Ti-substituted tunnel-type Na0.44MnO2oxide as a negative electrode for aqueous sodium-ion batteries The aqueous sodium-ion battery system is a safe and low-cost solution for large-scale energy storage, because of the abundance of sodium and inexpensive aqueous electrolytes. Although several positive electrode materials, for example, Na 0.44 MnO 2 , were proposed, few negative electrode materials, for example, activated carbon and NaTi 2 (PO 4 ) 3 , are available. Here we show that Ti-substituted Na 0.44 MnO 2 (Na 0.44 [Mn 1-x Ti x ]O 2 ) with tunnel structure can be used as a negative electrode material for aqueous sodium-ion batteries. This material exhibits superior cyclability even without the special treatment of oxygen removal from the aqueous solution. Atomic-scale characterizations based on spherical aberration-corrected electron microscopy and ab initio calculations are utilized to accurately identify the Ti substitution sites and sodium storage mechanism. Ti substitution tunes the charge ordering property and reaction pathway, significantly smoothing the discharge/charge profiles and lowering the storage voltage. Both the fundamental understanding and practical demonstrations suggest that Na 0.44 [Mn 1-x Ti x ]O 2 is a promising negative electrode material for aqueous sodium-ion batteries. Renewable energies such as solar and wind powers are being developed rapidly these days, critically demanding the development of large-scale energy storage in order to smooth the integration of their energies into the grid and improve the grid’s reliability. The electrochemical approach, with the flexibility, high energy conversion efficiency and simple maintenance, is one of the most promising means to store electricity in large scale among the various energy storage technologies [1] , [2] . Although lithium-ion batteries have been widely used in portable electronic devices and are considered to be the best choice for electric vehicles, the increasing cost and limited resources of lithium may restrict their application in large-scale energy storage systems [3] , [4] , [5] . Sodium-ion batteries have attracted extensive attentions for such large-scale applications in both scientific and technological aspects because of the abundance of sodium resources and potential low cost as well as the similarity of sodium-ion storage device to those of as lithium-ion batteries [6] , [7] , [8] , [9] , [10] , [11] , [12] , [13] , [14] , [15] , [16] , [17] , [18] , [19] , [20] . In particular, aqueous sodium-ion batteries have attracted great interest in terms of their safety, low-cost and high-rate capability [21] , [22] , [23] , [24] , [25] , [26] , [27] , [28] . Many interesting electrode materials have been studied in aqueous electrolytes. For the positive electrode materials, Prussian blue analogues, polyanionic compounds and oxides are widely investigated. Among the numerous identified oxides of potential interest, Na 0.44 MnO 2 with a tunnel structure is particularly attractive because of its unique large tunnels suitable for sodium insertion/extraction [29] , [30] , [31] , [32] , [33] , [34] . The crystal structure of Na 0.44 MnO 2 is shown in Fig. 1 . There are five crystallographic sites for manganese, where Mn(1), Mn(3) and Mn(4) sites are occupied by Mn 4+ , whereas Mn(2) and Mn(5) sites are occupied by Mn 3+ , exhibiting a charge ordering [35] . The framework is built up based on double and triple rutile-type chains of edge-sharing MnO 6 octahedra and single chains of corner-sharing MnO 5 . Three different types of sodium sites have been found within the tunnels formed by MnO 6 and MnO 5 polyhedrons. Two sodium sites (Na(2) and Na(3)) are situated in large S-shaped tunnels, whereas another site (Na(1)) is located in smaller tunnels. Unlike most layered oxides, Na 0.44 MnO 2 is very stable in aqueous solution even upon Na extraction and insertion [21] , [26] , [31] . For the negative electrode materials, only a few materials, including activated carbon and NaTi 2 (PO 4 ) 3 have been identified in the literature [21] , [26] , [27] , [28] for sodium-ion batteries. Although activated carbon for aqueous sodium-ion batteries is quite stable, the capacity is only ca. 30 mAh g −1 at a current rate of 1C and the cost is relatively high [36] . Sodiated NaTi 2 (PO 4 ) 3 suffers from sensitivity to oxygen in aqueous solution [37] . 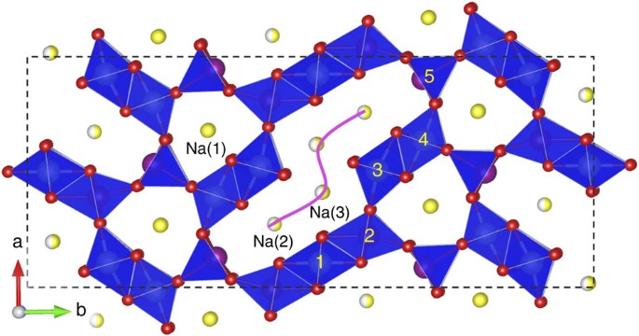Figure 1: Crystal structure of Na0.44MnO2. General view alongc-axis showing five crystallographic sites for manganese and three sites for sodium. Figure 1: Crystal structure of Na 0.44 MnO 2 . General view along c -axis showing five crystallographic sites for manganese and three sites for sodium. Full size image Here, we demonstrate that Ti-substituted Na 0.44 MnO 2 (Na 0.44 [Mn 1- x Ti x ]O 2 ( x =0.11, 0.22, 0.33, 0.44, 0.56) can be used as a negative electrode material in aqueous sodium-ion batteries with very stable cycling performance. The site occupancy of substituted Ti in the crystal structure is clearly demonstrated on an atomic scale and the sodium storage mechanism is revealed by multiple advanced characterization techniques. Structure of Na 0.44 [Mn 1- x Ti x ]O 2 The Na 0.44 [Mn 1- x Ti x ]O 2 series compounds were prepared by a simple solid-state reaction method using Na 2 CO 3 , Mn 2 O 3 and TiO 2 as precursors. Laboratory X-ray diffraction (XRD) patterns (Cu Kα radiation) of the as-prepared samples are shown in Fig. 2a . It can be seen that Ti-substituted Na 0.44 [Mn 1- x Ti x ]O 2 ( x =0.11, 0.22, 0.33, 0.39, 0.44, 0.56) maintain a crystal structure similar to their parent structure of Na 0.44 MnO 2 (bottom curve in Fig. 2a ). Further Rietveld refinements of the as-collected synchrotron XRD patterns are shown in Fig. 2b,c and Supplementary Fig. 1 . Major diffraction peaks can be indexed with space group of Pbam . (Note that some minor impurities were found in some substituted samples, which we were unable to index.) [38] Lattice parameter evolution of Na 0.44 [Mn 1- x Ti x ]O 2 ( x =0.17, 0.22, 0.34, 0.39, 0.56) is shown in Supplementary Table 1 . It can be seen that lattice parameters a and c (slightly) expand as Ti concentration increases, whereas lattice parameter b first expands ( x ≤0.34) and then shrinks. The unit cell volume was found to expand as a result of Ti substitution. The morphology of the sample was revealed as a rod-like shape with a length of ca. 10 μm and a diameter of ca. 1 μm by scanning electron microscopy (SEM) observation as shown in the Supplementary Fig. 2 . A combination of the characterization tools, including synchrotron-based powder XRD, and scanning transmission electron microscopy (STEM) were used, together with density functional theory (DFT) calculation, to locate the potential Ti atomic positions in the as-prepared compounds. In fact, tunnel-type Na 0.44 MnO 2 oxide has been widely studied as a potential positive electrode for rechargeable sodium-ion or lithium-ion (after Na + /Li + ion exchange) batteries [30] , [31] , [32] , [35] , [39] . Although the Ti-substituted single crystal of ‘Na 4 [Mn 4 Ti 5 ]O 18 ’ was firstly reported by Mumme as early as 1968 (ref. 40 ), the structure of this phase has still not been well understood, after several decades. Doeff et al. synthesized a series of Na 0.44 [Mn 1- x Ti x ]O 2 (0< x <0.56) in powder form, and suggested that Ti may potentially replace Mn at all four MnO 6 octahedra sites but not at the Mn at the MnO 5 square pyramid site, based on a bonding environment argument [38] . However, the accurate Ti and Mn site occupancies were not clearly identified through quantitative XRD analysis in that work. This motivated us to explore the accurate crystal structure of these Ti-substituted Na 0.44 [Mn 1- x Ti x ]O 2 further by using high-resolution synchrotron XRD. Interestingly, we noticed very strong anisotropic peak broadening character of all the collected diffraction patterns, as exemplified by the much broader (140) diffraction peak; this phenomenon has also been observed in Na 0.44 MnO 2 (ref. 41 ). It was found that an anisotropic size-related broadening term was needed to effectively model the as-collected diffraction patterns [42] . The refined crystal structure is similar to the one shown in Fig. 1 , whereas the occupation of transition metals is displayed in Table 1 . It was revealed that Ti ions first replace Mn at Mn(3) and Mn(4) sites at a low substitution amount (when x is 0.17, 0.22), and further replace Mn at the Mn(1) site as x increases to 0.34 and 0.39. When the nominal x =0.56, Ti was found to mainly occupy Mn(1), Mn(3) and Mn(4) sites. In addition, Mn(2) sites were also found to be slightly occupied by Ti. These findings are in good agreement with DFT calculations ( Fig. 2e ). Such calculations show representative configurations of Na 0.44 [Mn 0.44 Ti 0.56 ]O 2 , indicating that the preferred occupancies of Ti at Mn(1), Mn(3) and Mn(4) offer the most stable configurations of transition metals in the structure. On the other hand, other types of Ti doped-configurations in Mn sites can destabilize the structure by as much as 126 meV per formula unit (f.u.). In contrast, it was noted that a partial Ti occupation in Mn(2) site (instead of Mn(1) site), as shown in the first two configurations ( Fig. 2d ), destabilizes the structure only by 24 meV per f.u. Considering the thermal energy scale of ~25 meV per f.u. at room temperature, this energy barrier is too small to restrict the possibility of the partial Ti occupancy of the Mn(2) site, especially for materials synthesized via a high-temperature route. 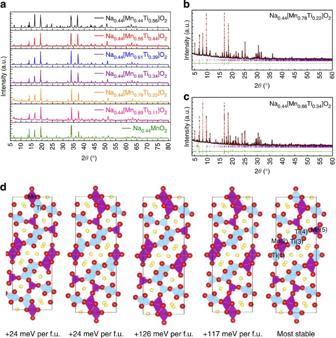Figure 2: Structure of Na0.44[Mn1-xTix]O2. (a) XRD patterns of Na0.44[Mn1-xTix]O2compounds prepared at 950 °C, arranged in order of increasing titanium content from bottom to top. The bottom pattern is that of Na0.44MnO2. (b) The Rietveld plot (λ=0.7785 Å) for refined Na0.44[Mn0.78Ti0.22]O2synchrotron XRD pattern with experimental data in black dots, calculated curve in red and difference curve in olive. (c) The Rietveld plot (λ=0.7785 Å) for refined Na0.44[Mn0.66Ti0.34]O2pattern with experimental data in black dots, calculated curve in red and difference curve in olive. (d) General view of the crystal structure and view alongc-axis showing sites for Mn ions and Ti ions located in MnO6/TiO6octahedral/square pyramid. The cyan octahedral represents TiO6, whereas purple one represents MnO6/MnO5polyhedron. Detailed information can be found in Supplementary Table 2 . It should be noted that the chemical formulas of the materials used in this communication are nominal stoichiometry based on the contents of the starting materials in synthesis. The actual chemical stoichiometry in Na 0.44 [Mn 1- x Ti x ]O 2 phase can be estimated from the XRD refinement results shown in Table 1 . According to the refinement result, the maximum Ti substitution amount is around 0.44 in Na 0.44 MnO 2 . It was also found that Na at the Na(1) site was not fully occupied, but exhibited an occupancy range between 0.7 and 0.8 for the as-prepared samples, whereas occupancy at the Na(2) and Na(3) sites was found to be slightly higher than the ideal occupancy of 0.5; thus the total Na was found to be slightly less than the nominal 0.44. Figure 2: Structure of Na 0.44 [Mn 1- x Ti x ]O 2 . ( a ) XRD patterns of Na 0.44 [Mn 1- x Ti x ]O 2 compounds prepared at 950 °C, arranged in order of increasing titanium content from bottom to top. The bottom pattern is that of Na 0.44 MnO 2 . ( b ) The Rietveld plot ( λ =0.7785 Å) for refined Na 0.44 [Mn 0.78 Ti 0.22 ]O 2 synchrotron XRD pattern with experimental data in black dots, calculated curve in red and difference curve in olive. ( c ) The Rietveld plot ( λ =0.7785 Å) for refined Na 0.44 [Mn 0.66 Ti 0.34 ]O 2 pattern with experimental data in black dots, calculated curve in red and difference curve in olive. ( d ) General view of the crystal structure and view along c -axis showing sites for Mn ions and Ti ions located in MnO 6 /TiO 6 octahedral/square pyramid. The cyan octahedral represents TiO 6 , whereas purple one represents MnO 6 /MnO 5 polyhedron. Full size image Table 1 Mn/Ti occupancy in the Na 0.44 [Mn 1- x Ti x ]O 2 from synchrotron XRD Rietveld refinements. Full size table To further confirm this result, advanced spherical aberration-corrected electron microscopy experiments were performed to determine the structure at atomic scale ( Fig. 3 ). The high-angle annular dark field (HAADF) images of the pristine Na 0.44 [Mn 0.44 Ti 0.56 ]O 2 recorded along the [001], [010] and [100] zone axes are shown in Fig. 3b and Supplementary Fig. 3 . The contrast of the HAADF image exhibits an approximately Z 1.7 dependence with respect to the atomic number Z ; therefore the brighter dots represent the heavier atomic columns (Ti and Mn) [43] . The atomic arrangement revealed in the HAADF image is identical to the simulated atomic configuration viewed along [001] orientation ( Fig. 3a ). The large S-shaped tunnel and small hexagonal tunnel formed by MO 6 and MO 5 polyhedrons can be clearly seen, with Na atoms filled in. Therefore, the five different transition metal sites and three sodium sites are clearly distinguished in the image. The Ti and Mn site preferences were further examined by atomic-scale STEM-electron energy loss spectrum (EELS). The line scanning was performed on the selected area marked with a red rectangle, as shown on the HAADF image, where Ti and Mn EELS spectra were collected simultaneously ( Fig. 3c ). The bright dots shown on the projection view of the stacked EELS spectra represent the excitation of the EELS signal for the corresponding elements therein, while the contrast represents its relative content. It can be deduced that Mn(1), Mn(3) and Mn(4) sites are filled with Ti atoms, whereas the Mn(2) site is much less filled with Ti atoms, as indicated by the low contrast shown on the Ti EELS image. No Ti EELS signal can be seen on the Mn(5) site, which indicates that the Mn(5) site is fully occupied with Mn atoms. Manganese EELS signals are observed on all transition metal sites. Therefore, it can be concluded that the Mn(5) site is solely occupied by Mn atoms, whereas Mn(1), Mn(2), Mn(3) and Mn(4) sites are filled by Mn and Ti atoms with different ratios. Atomic-scale energy dispersive spectroscopy (EDS) of Na 0.44 [Mn 0.44 Ti 0.56 ]O 2 was also carried out to confirm the elemental distribution, the corresponding elemental mappings of Mn, Ti and Na are exhibited in Fig. 3e–g , respectively. It can be seen that the Mn(5) site is fully occupied by Mn, while other sites are taken up by a mixture of Mn and Ti. Furthermore, Mn(1), Mn(3) and Mn(4) sites are mainly occupied by Ti, whereas the Mn(2) site is mainly occupied by Mn. These results agree well with the refinement results, DFT calculations and EELS outcomes. This disordered Mn/Ti arrangement is in sharp contrast with the single-crystal structure of Na 0.44 [Mn 0.44 Ti 0.56 ]O 2 , with its ordered Mn/Ti arrangement [40] . 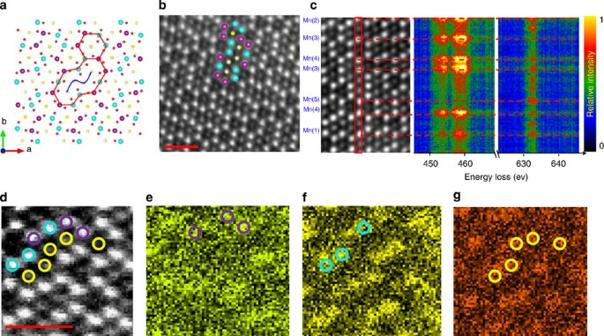Figure 3: STEM imaging. (a) General view of the crystal structure and view along [001] zone axis. (b) HAADF-STEM image for the as-prepared Na0.44[Mn0.44Ti0.56]O2materials along [001] zone axis. Scale bar, 1 nm. (c) The EELS image of Na0.44[Mn0.44Ti0.56]O2. The energy dispersive spectroscopy mapping, (d) HAADF-STEM image, (e–g) the corresponding elemental mapping of the Mn, Ti and Na elements, respectively. Scale bar, 1 nm. Figure 3: STEM imaging. ( a ) General view of the crystal structure and view along [001] zone axis. ( b ) HAADF-STEM image for the as-prepared Na 0.44 [Mn 0.44 Ti 0.56 ]O 2 materials along [001] zone axis. Scale bar, 1 nm. ( c ) The EELS image of Na 0.44 [Mn 0.44 Ti 0.56 ]O 2 . The energy dispersive spectroscopy mapping, ( d ) HAADF-STEM image, ( e – g ) the corresponding elemental mapping of the Mn, Ti and Na elements, respectively. Scale bar, 1 nm. Full size image Sodium storage performance in non-aqueous system The sodium storage performance of Na 0.44 [Mn 1- x Ti x ]O 2 ( x =0, 0.11, 0.22, 0.33, 0.44, 0.56) in non-aqueous media was tested with Na 0.44 [Mn 1- x Ti x ]O 2 |Na half cells. On the basis of the above-described structural characteristics, the Na(2) and Na(3) sites located in the S-shaped tunnels are reversibly accessible, whereas the sodium ions located on the Na(1) site are not, or are hardly extracted. It is therefore expected that the achievable composition is Na 0.22 [Mn 1- x Ti x ]O 2 during Na extraction, while full occupancy of all the sodium sites gives a composition of Na 0.66 [Mn 1- x Ti x ]O 2 during Na insertion. 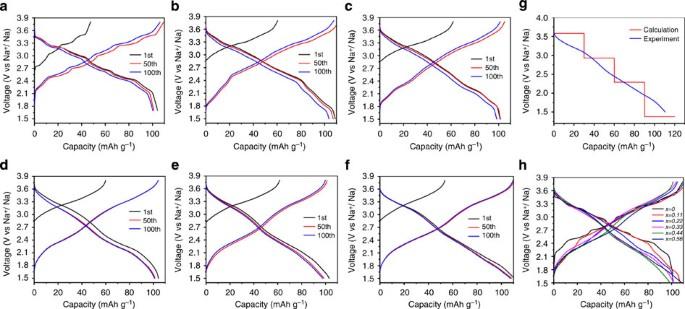Figure 4: Sodium storage performance of Na0.44[Mn1-xTix]O2electrodes in non-aqueous solution. The 1st, 50th and 100th discharge/charge curves at a current rate of C/10 in the voltage range of 1.5 and 3.8 V versus Na+/Na. (a) Na0.44MnO2, (b) Na0.44[Mn0.89Ti0.11]O2, (c) Na0.44[Mn0.78Ti0.22]O2, (d) Na0.44[Mn0.67Ti0.33]O2, (e) Na0.44[Mn0.56Ti0.44]O2, (f) Na0.44[Mn0.44Ti0.56]O2. (g) Comparison of DFT calculated voltage curve and experiment curve for the Nax[Mn0.44Ti0.56]O2electrode (note that entropy and temperature effects were not considered in calculation). (h) Comparison of the 2nd charge/discharge curve for Na0.44[Mn1-xTix]O2. Figure 4a–f shows the charge and discharge curves recorded under a current rate of 0.1C (12.6 mA g −1 ) cycling in the voltage range of 1.5–3.9 V. The observed first charge capacity is about 45–60 mAh g −1 and the subsequent reversible discharge/charge capacity is about 100–110 mAh g −1 for all samples, in good agreement with the structural estimation for the Na composition (Na 0.22 to Na 0.66 ). (Note that the discharge capacity is larger than the first charge capacity, which is due to the additional Na insertion below 2.7 V) Multiple plateaus were observed during Na extraction/insertion for the un-substituted Na 0.44 MnO 2 , a phenomenon related to a series of phase transitions (Na + /vacancy ordering and/or charge ordering), as interpreted in previous earlier literature [35] , [41] . With an increase of Ti substitution, the multiple plateaus on the voltage profile gradually turn into a sloping feature, in analogy to our recent observation of Na 0.66 [Li 0.22 Ti 0.78 ]O 2 negative electrode material (Li substituted NaTiO 2 ) [44] . This behaviour could be caused by the disordered Mn/Ti arrangement, which breaks the charge ordering and/or Na + /vacancy ordering. The experimentally observed Na storage voltage is consistent with the average value (~2.5 V) predicted from the DFT calculations shown in Fig. 4g . The stepwise feature of the voltage profile from the calculations is not due to the phase transition, but instead, is due to the finite number of intermediate compositions that we took account of in the computations. The ordered model due to the finite size of supercells as shown in Fig. 2d produces the artificial long-range Na + /vacancy ordering and/or charge ordering. An infinite number of compositional computations would result in a sloping voltage profile. In this regard, the formation energy of Na x [Mn 0.44 Ti 0.56 ]O 2 was found to follow a typical convex hull type of the solid solution as shown in Supplementary Fig. 4 . These data support the notion that the Na insertion/extraction into/from Na x [Mn 0.44 Ti 0.56 ]O 2 is based on a solid-solution reaction in a range of 0.22< x <0.66. Furthermore, when compared with the un-substituted Na 0.44 MnO 2 sample, it is interesting to find in Fig. 4h that the discharge voltage above 2.8 V are similar for both samples, whereas for Ti-substituted samples, the discharge voltages below 2.8 V are ca. 0.2 V in average lower than those of the un-substituted sample. The lower average Na storage voltage of the Ti-substituted samples extends their potential application as negative electrodes for sodium-ion batteries. Figure 4: Sodium storage performance of Na 0.44 [Mn 1- x Ti x ]O 2 electrodes in non-aqueous solution. The 1st, 50th and 100th discharge/charge curves at a current rate of C/10 in the voltage range of 1.5 and 3.8 V versus Na + /Na. ( a ) Na 0.44 MnO 2 , ( b ) Na 0.44 [Mn 0.89 Ti 0.11 ]O 2 , ( c ) Na 0.44 [Mn 0.78 Ti 0.22 ]O 2 , ( d ) Na 0.44 [Mn 0.67 Ti 0.33 ]O 2 , ( e ) Na 0.44 [Mn 0.56 Ti 0.44 ]O 2 , ( f ) Na 0.44 [Mn 0.44 Ti 0.56 ]O 2 . ( g ) Comparison of DFT calculated voltage curve and experiment curve for the Na x [Mn 0.44 Ti 0.56 ]O 2 electrode (note that entropy and temperature effects were not considered in calculation). ( h ) Comparison of the 2nd charge/discharge curve for Na 0.44 [Mn 1- x Ti x ]O 2 . Full size image Sodium storage performance in aqueous system The Na storage behaviours revealed in non-aqueous media indicate that these materials may be applicable to aqueous media system with remarkable reversibility and suitable operating voltage. The cyclic reversibility of these materials was first examined in non-aqueous media in a narrow voltage range of 1.8–2.8 V versus Na + /Na ( Supplementary Figs 5 and 6 ), which fits with the operating voltage for negative electrodes in aqueous media (−0.6 to 0 V versus saturated calomel electrode (SCE)). The capacity retentions for both Na 0.44 MnO 2 and Na 0.44 [Mn 0.44 Ti 0.56 ]O 2 are higher than 96% after 1,100 cycles ( Supplementary Fig. 5 ), indicating ultra-high structural stability during Na insertion and extraction. The Na storage performance of the Na 0.44 MnO 2 and Na 0.44 [Mn 0.44 Ti 0.56 ]O 2 in aqueous media is shown in Fig. 5 . Overall, the discharge–charge voltage profiles are similar to that observed in non-aqueous media. The voltage plateaus on the charge–discharge curve of Na 0.44 MnO 2 measured in aqueous media are not as obvious as those recorded in non-aqueous media, probably due to the existence of pseudo-capacitance from the redox reactions and double-layer electric capacitance as well as the higher C-rate adopted during aqueous measurements [45] . The polarization between discharge and charge of the Na 0.44 [Mn 0.44 Ti 0.56 ]O 2 electrode is around 50 mV ( Supplementary Fig. 7 ), which is somehow slightly smaller than that of un-substituted Na 0.44 MnO 2 electrode, although Na 0.44 MnO 2 exhibits higher electronic conductivity than Ti-substituted samples [46] . This indicates that Na + ion diffusion might be the limiting step. Stable capacities of 32 and 37 mAh g −1 can be obtained for Na 0.44 MnO 2 and Na 0.44 [Mn 0.44 Ti 0.56 ]O 2 charge–discharged at 2C rate, respectively, which is higher than that of activated carbon shown in Supplementary Fig. 8 . These materials also demonstrate excellent cycling performance with no evident capacity fading after 400 cycles, even without taking special caution to remove the oxygen in the aqueous solution. It is known that the existence of the O 2 in the aqueous system will react with the discharged electrodes, resulting in deteriorated electrochemical cycle performances. However, it has been reported that the Na 0.44 MnO 2 can function as an electrocatalyst for oxygen reduction reaction in rechargeable Li-O 2 batteries [47] . In this sense, the electrode itself is stable when a small amount of O 2 exists. The superior electrochemical performance demonstrates that these materials can be used as negative electrode materials for aqueous sodium-ion battery applications. 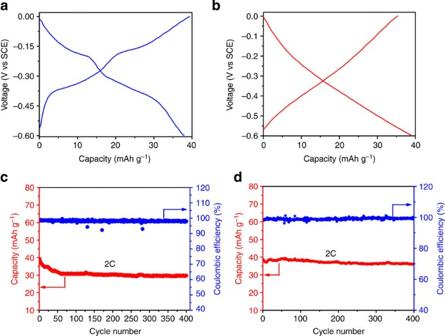Figure 5: Sodium storage performance of Na0.44[Mn1-xTix]O2negative electrodes in aqueous solution. The 1st discharge/charge curves in the voltage range of −0.6 and 0 V versus SCE for (a) Na0.44MnO2electrode and (b) Na0.44[Mn0.44Ti0.56]O2electrode at a current rate of 2C. Long-term cycling performance for (c) Na0.44MnO2electrode and (d) Na0.44[Mn0.44Ti0.56]O2at a current rate of 2C. Figure 5: Sodium storage performance of Na 0.44 [Mn 1- x Ti x ]O 2 negative electrodes in aqueous solution. The 1st discharge/charge curves in the voltage range of −0.6 and 0 V versus SCE for ( a ) Na 0.44 MnO 2 electrode and ( b ) Na 0.44 [Mn 0.44 Ti 0.56 ]O 2 electrode at a current rate of 2C. Long-term cycling performance for ( c ) Na 0.44 MnO 2 electrode and (d) Na 0.44 [Mn 0.44 Ti 0.56 ]O 2 at a current rate of 2C. Full size image To further understand the structural changes in Na 0.44 [Mn 0.44 Ti 0.56 ]O 2 during Na insertion and extraction, an in situ XRD experiment was performed, and the results are presented in Fig. 6a . Most of the XRD reflections (for example, (040), (130), (140)) reveal continuous peak shift during Na insertion/extraction. There is no evident appearance of a new phase upon Na insertion/extraction into/from Na 0.44 [Mn 0.44 Ti 0.56 ]O 2 in a wide Na content range. Although a significant amount of Mn 3+ was reserved in Na 0.44 [Mn 0.44 Ti 0.56 ]O 2 structure for the entire range of electrochemical cycles, the main crystal structure was maintained during the entire charge/discharge process without any obvious structure transformation. This is further supported by the ex situ STEM results shown in Supplementary Fig. 9 , revealing that the framework of transition metal arrangement was well retained after Na extraction and insertion. Interestingly, a visible biphasic region can be observed at the end of the discharge process, which is probably due to the smaller unit cell volume of Na 0.44 [Mn 0.44 Ti 0.56 ]O 2 compared with Na 0.66 [Mn 0.44 Ti 0.56 ]O 2 , and the slow kinetics of the phase transition [35] . All of the XRD patterns recorded during the in situ investigations have been refined (full patterns are shown in Supplementary Fig. 10 ). From the evolution of the lattice parameters, Vegard’s law is verified in general, within the regions separated by the dashed line in Fig. 6b . (Evolution of the unit cell volume is shown in Supplementary Fig. 11 .) At two-phase transition range, if it exists, may occur only in narrow regions across the dashed line. These observations are in good agreement with the charge–discharge profile. Overall, it is most likely that the phase transition may proceed through several solid-solution reactions during Na insertion/extraction into/from Na 0.44 [Mn 0.44 Ti 0.56 ]O 2 , different from the significant consecutive two-phase reaction behaviour observed in Na 0.44 MnO 2 (ref. 41 ). As interpreted in previous work, the major ‘ a ’ and ‘ b ’ lattice changes can be directly linked to the Mn 3+ /Mn 4+ redox reaction at specific Mn sites (for example, Mn(2) site relates to ‘ b ’ and Mn(3) site relates to ‘ a ’), owing to the Jahn-Teller effect as well as different orientations of the Mn-O octahedron in structure [35] . Ti substitution induces significant Ti/Mn mixing in all octahedral sites. As Ti ions will remain at Ti 4+ at all sites, it is expected that the valance states of Mn at each site may be altered in comparison with that of Na 0.44 MnO 2 in order to keep charge neutrality. This could cause different Mn 3+ /Mn 4+ redox reaction mechanisms at each individual Mn site, leading to a different lattice change manner when compared with Na 0.44 MnO 2 . 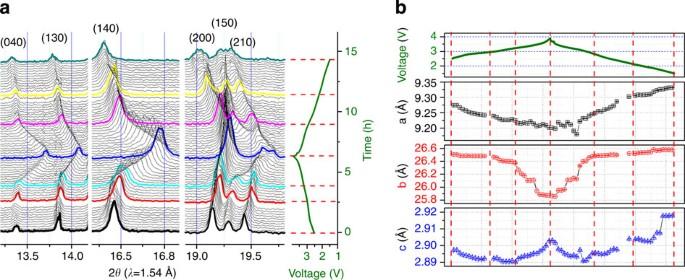Figure 6: Structure evolution upon Na extraction/insertion. (a)In situXRD patterns collected during the first discharge/charge of the Na/Na0.44[Mn0.44Ti0.56]O2cell under a current rate of C/10 at a voltage range between 1.5 and 3.9 V. For easy comparison with results in the literature, the 2θangle has been converted to values corresponding to the more common laboratory Cu Ka radiation (χ=1.54 Å). (b) Evolution of the Lattice parameters during charge/discharge process. Figure 6: Structure evolution upon Na extraction/insertion. ( a ) In situ XRD patterns collected during the first discharge/charge of the Na/Na 0.44 [Mn 0.44 Ti 0.56 ]O 2 cell under a current rate of C/10 at a voltage range between 1.5 and 3.9 V. For easy comparison with results in the literature, the 2 θ angle has been converted to values corresponding to the more common laboratory Cu Ka radiation ( χ =1.54 Å). ( b ) Evolution of the Lattice parameters during charge/discharge process. Full size image In situ Mn K-edge X-ray absorption spectroscopy (XAS) spectra were collected to examine the variations of the oxidation states during electrochemical cycling. The corresponding X-ray absorption near edge spectroscopy (XANES) results are shown in Fig. 7a . An entire edge shift of the XANES spectra can be observed during the charge and discharge process, which represents a redox reaction of Mn ions for the entire electrochemical cycle. To semi-quantitatively determine the oxidation states of Mn, the evolution of the edge energy of the XANES spectra was plotted in Fig. 7b along with Mn 2 O 3 (Mn 3+ ) as reference. The average oxidation state of Mn, changes from around +3 in the pristine material towards a higher value (<+4) during the charge process. During discharge, Mn ions are continually reduced, and the average oxidation state of Mn is lower than +3 at the fully discharged state. The ex situ Mn XANES results further confirm the charge compensation mechanism of Mn. Owing to the strong absorption from other components of the in situ cell and the lower K-edge energy nature of Ti, it is difficult to perform an in situ Ti K-edge XAS experiment. Therefore, ex situ Ti K-edge XANES spectra were collected at selected charge and discharge states as shown in Fig. 7c . All spectra remain at the same edge position as the reference material Li 4 Ti 5 O 12 , indicating Ti ions remain at Ti 4+ during the entire charge/discharge process. The charge compensations can be concluded to take place solely on Mn ions. In addition, as it is generally accepted that the square pyramidal Mn(5) site will remain at the Mn 3+ state during Na insertion/extraction [35] , a portion of the Mn ions on other sites should be reduced to Mn 2+ to match the observed discharge capacity in Na 0.44 [Mn 0.44 Ti 0.56 ]O 2 . This differs from the observation of Na 0.44 MnO 2 , where Mn 3+ /Mn 4+ redox reaction on Mn(2) and Mn(3) sites can compensate the charge during the entire Na extraction/insertion process. The site preference of the Mn 2+ in the discharged Na 0.44 [Mn 0.44 Ti 0.56 ]O 2 will be further interpreted by DFT calculation in the following discussion. 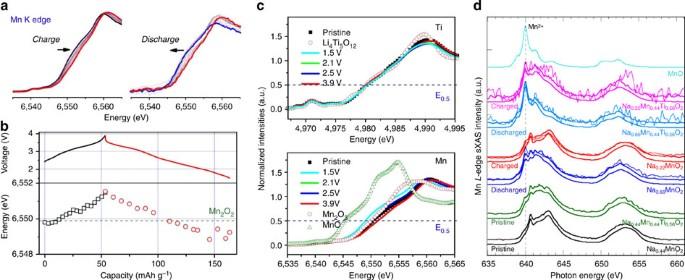Figure 7: Charge compensation mechanism upon Na extraction/insertion in Na0.44[Mn0.44Ti0.56]O2. (a)In situXANES spectra at Mn K-edge collected during initial charge and discharge at a current rate of C/8 between 1.5 and 3.9 V voltage range (data are obtained in two differentin situcells for charge and discharge process separately). (b) Variation of Mn K-edge position during initial charge and discharge. (c) Ti and Mn K-edge XANES spectraex situcollected at different charge/discharge states. Spectra of reference materials were represented for comparison. (d) MnL-edge sXAS spectra collected on Nax[Mn0.44Ti0.56]O2samples in comparison with that of NaxMnO2(x=0.22, 0.44 and 0.66). The spectra of chemically prepared samples are shown in thick solid lines, whereas those of electrochemically prepared ones are in thin dot lines. The calculated spectra (thick dash lines) using the linear combination of the Mn2+, Mn3+and Mn4+reference spectra agree well with experiments. Figure 7: Charge compensation mechanism upon Na extraction/insertion in Na 0.44 [Mn 0.44 Ti 0.56 ]O 2 . ( a ) In situ XANES spectra at Mn K-edge collected during initial charge and discharge at a current rate of C/8 between 1.5 and 3.9 V voltage range (data are obtained in two different in situ cells for charge and discharge process separately). ( b ) Variation of Mn K-edge position during initial charge and discharge. ( c ) Ti and Mn K-edge XANES spectra ex situ collected at different charge/discharge states. Spectra of reference materials were represented for comparison. ( d ) Mn L -edge sXAS spectra collected on Na x [Mn 0.44 Ti 0.56 ]O 2 samples in comparison with that of Na x MnO 2 ( x =0.22, 0.44 and 0.66). The spectra of chemically prepared samples are shown in thick solid lines, whereas those of electrochemically prepared ones are in thin dot lines. The calculated spectra (thick dash lines) using the linear combination of the Mn 2+ , Mn 3+ and Mn 4+ reference spectra agree well with experiments. Full size image Soft XAS (sXAS) enables us to study the evolution of the manganese oxidation states on the electrode surface with higher energy resolution. Mn L -edge sXAS offers a direct probe of the Mn 3 d electrons through dipole-allowed 2 p -to-3 d transition. Compared with the hard X-ray spectroscopy, sXAS is more surface sensitive with a probing depth of around several nanometres if the total electron yield is measured. Figure 7d shows Mn L -edge sXAS spectra collected on pristine Na 0.44 MnO 2 and Na 0.44 [Mn 0.44 Ti 0.56 ]O 2 powder samples, as well as on both chemically and electrochemically prepared Na x MnO 2 and Na x [Mn 0.44 Ti 0.56 ]O 2 powder and electrode samples with nominally x =0.22 and 0.66. The spectra consist of well-separated absorption features in two regions, L 2 (638–646 eV) and L 3 (649–656 eV), resulting from the 2p core-hole spin-orbital splitting. In general, manganese compounds with manganese ions of the same oxidation state in the octahedral crystal field display similar Mn L -edge sXAS spectra in spite of their different compositions and crystal structures. Although for those with different manganese oxidation states, dramatically different absorption features are observed and the overall absorption intensity shifts to higher photon energy along with the increased manganese oxidation states. This enables us to quantitatively analyse the evolution of the manganese oxidation states in complex battery material. As shown in Fig. 7d , the calculated spectra (thick dashed lines) using the linear combination of the Mn 2+ , Mn 3+ and Mn 4+ reference spectra agree well with the experiments. The fitting results of the proportions of Mn 2+ , Mn 3+ and Mn 4+ in each sample are shown in Supplementary Table 3 . The Mn- L sXAS spectrum of the as-prepared Na 0.44 MnO 2 powder displays 42% Mn 3+ and 58% Mn 4+ , which are very close to its nominal values (44% Mn 3+ and 56% Mn 4+ ). The Ti substitution reduces the manganese oxidation states, so around 67% Mn 3+ and 31% Mn 4+ are found in the as-prepared Na 0.44 [Mn 0.44 Ti 0.56 ]O 2 powder, which is also evidenced by the increased lower-energy absorption intensity in the raw data ( Fig. 7d ). As the maximum Ti substitution amount is around 0.44 in nominal Na 0.44 [Mn 0.44 Ti 0.56 ]O 2 , there would be a small amount of Mn 4+ (0.12) to keep the charge neutrality. After Na insertion (Na 0.66 ), a sharp absorption peak associated with Mn 2+ is observed at 640 eV in both samples, with and without Ti-substituted ion (Na 0.66 MnO 2 and Na 0.66 [Mn 0.44 Ti 0.56 ]O 2 ), which suggests the insertion of Na could reduce the oxidation state of the manganese ions down to Mn 2+ . In particular, the Mn 2+ concentration in Na 0.66 [Mn 0.44 Ti 0.56 ]O 2 reaches as high as 60%. Note that the electrochemically prepared samples display sXAS spectra similar to those of the chemically prepared ones, but with a much weaker signal, especially for the Ti-substituted samples. As sXAS is a surface-sensitive technique, this result indicates the deficiency of manganese ions on the electrode surface, which may be related to the possible changes of the surface structure. Unlike hard X-ray results, the sXAS obtained in samples after Na extraction (Na 0.22 MnO 2 and Na 0.22 [Mn 0.44 Ti 0.56 ]O 2 ) shows the manganese ions on the sample surface are reduced compared with the pristine (Na 0.44 ) samples. It is, however, consistent with our previous observation in LiNi 0.5 Mn 1.5 O 4 (ref. 48 ). The reduced manganese oxidation state observed in sXAS stems from the surface catalytic reaction and is enhanced by the large surface area of the nanoparticles. The presence of Mn 2+ in the sodiated sample (Na 0.66 [Mn 0.44 Ti 0.56 ]O 2 ) is further supported by DFT calculations as shown in Fig. 8 . It can be seen from Fig. 8 that the Mn 3+ at the Mn(2) site is reduced to Mn 2+ upon Na insertion. This situation differs from the Na 0.44 MnO 2 sample where Mn 4+ at Mn(3) site is reduced to Mn 3+ , which is reflected by a higher discharge voltage during Na insertion (Mn 4+ /Mn 3+ redox) as indicated by DFT calculations [35] . On the basis of the above discussion combined with XAS results, we can conclude that upon Na insertion into Na 0.44 [Mn 0.44 Ti 0.56 ]O 2 , the residual Mn 4+ ions at Mn(3) sites are first reduced to Mn 3+ , and then Mn 3+ ions at Mn(2) sites are further reduced to Mn 2+ . Upon Na extraction from Na 0.44 [Mn 0.44 Ti 0.56 ]O 2 , Mn 3+ ions at Mn(2) sites are oxidized into Mn 4+ . Ti substitution changes the charge compensation mechanism in Na 0.44 MnO 2 . 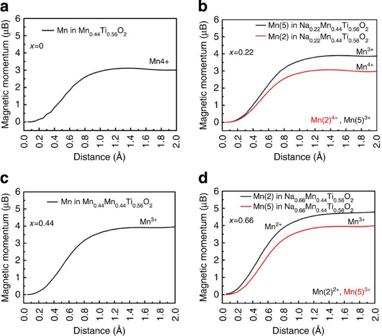Figure 8: DFT calculation. Valance state variation of Mn for Nax[Mn0.44Ti0.56]O2(a)x=0, (b)x=0.22, (c)x=0.44, (d)x=0.66. Figure 8: DFT calculation. Valance state variation of Mn for Na x [Mn 0.44 Ti 0.56 ]O 2 ( a ) x =0, (b) x =0.22, ( c ) x =0.44, ( d ) x =0.66. Full size image In summary, the tunnel-type Na 0.44 [Mn 1- x Ti x ]O 2 ( x =0, 0.11, 0.22, 0.33, 0.44, 0.56) show different charge/discharge curves with the increase of Ti content. In particular, Ti substitution can break the charge ordering, significantly smooth the discharge/charge curves and lower the storage voltage. The Ti occupancy in the crystal structure was also clearly demonstrated at atomic scale by high-resolution XRD, EELS and STEM EDS, in good agreement with the DFT calculations. It was found that Ti 4+ would first preferentially occupy the Mn(3) and, Mn(4) sites, and then the Mn(1) site with increasing Ti content, whereas the Mn(2) site would be slightly occupied by Ti and Mn(5) site remain unchanged. Upon sodium insertion or extraction, the oxidation states of Mn(5) and Ti remain unchanged, whereas Mn at the Mn(2) and Mn(3) sites would be responsible for the charge compensation. More interestingly, this material can be used as a negative electrode for aqueous sodium-ion batteries with very stable cycling performance. In addition to the promising application in aqueous sodium-ion batteries, these findings provide new insight for designing even better tunnel-type electrode materials for the development of rechargeable batteries for large-scale energy storage systems. Material synthesis The series of materials was prepared by a solid-state reaction method using precursors of Na 2 CO 3 (99%), Mn 2 O 3 and TiO 2 (99.5%, anatase form). An excess of 2 mol% Na 2 CO 3 was used to compensate for the Na loss during high-temperature synthesis. The starting materials were ground in an agate mortar and pressed into pellets under pressure of 20 MPa. Then the pellets were heated at 950 °C for 15 h in an alumina crucible to form the final products. Hard X-ray diffraction and absorption spectroscopy In situ and ex situ hard XAS experiments were performed at beamline X18A of the National Synchrotron Light Source in Brookhaven National Laboratory (NSLS, BNL) in transmission mode with a Si (111) double-crystal monochromator detuned to the 35–50% value of its original maximum intensity to eliminate the higher-order harmonics. Detailed in situ experimental configurations are reported in our previous paper [49] . The reference spectrum of each element was simultaneously collected with the corresponding spectrum of the in situ cells by using a reference metal foil. Energy calibration was carried out with the first inflection point of the K-edge spectrum of the reference metal foil (Ti: 4966, eV, Mn: 6539, eV). XANES was analysed by the ATHENA software package. Synchrotron XRD of powder samples were collected at beamline X14A (NSLS, BNL) with a 1D linear position sensitive detector at a distance of about 1.4 m to the sample centre and a wavelength of approximately 0.78 Å. Structures of Na 0.44 [Mn 1- x Ti x ]O 2 were refined using the Rietveld method as implemented in the TOPAS software package (Bruker-AXS, version 4.2), fundamental parameters are used to model the peak shape contribution from the instrument. To effectively model the strong anisotropic broadening peaks, a modified Peter Stephens’ anisotropic broadening function was utilized with the original strain broadening related term (~tan θ ) replaced by a size broadening related term (~1/cos θ ). During refinement, atomic displacement of Na, Mn and Ti was fixed, whereas all other parameters including atomic positions and site occupancies were refined simultaneously until the refinement converged. Structure of Na 0.44 [Mn 1- x Ti x ]O 2 was directly solved from synchrotron powder XRD data by using charge flipping method in Jana 2006 (superflip implemented). All atoms including O were successfully identified. This compound was found to have essential similar crystal structure as Na 0.44 [Mn 1- x Ti x ]O 2 compounds, however, almost no anisotropic peak broadening was found for this sample. Further Rietveld refinement was carried out in TOPAS 4.2 with similar procedure mentioned in the previous paragraph. Soft X-ray absorption spectroscopy The electrodes were electrochemically cycled to certain stages in coin cells. Afterwards, they were disassembled and the electrodes were rinsed with dimethyl carbonate (DMC) thoroughly and dried in vacuum to remove any residue. The Na 0.44 [Mn 0.44 Ti 0.56 ]O 2 powder was chemically sodiated [50] , [51] by chemical reduction with sodium-biphenyl-1,2-dimethoxyethane (DME) solution as sodiating reagent. In a typical process, 0.0543, g pure sodium was dissolved into 10 ml colourless 1 M biphenyl-DME solution, forming a dark-green organic solution as the sodiating reagent. Then, 1 g Na 0.44 [Mn 0.44 Ti 0.56 ]O 2 powder was immersed into this solution (corresponding to 0.22 mol Na per 1 mol Na 0.44 [Mn 0.44 Ti 0.56 ]O 2 ). The slurry was stirred until the colour of the solution fade completely to obtain the sodiated products. The products were washed by DME several times, and dried in the vacuum for overnight. Chemically sodium extraction of the sample was accomplished by reaction with a strong nitronium tetrafluoroborate (NO 2 BF 4 , Aldrich, 98%) [15] . Solid NO 2 BF 4 was dissolved in acetonitrile and Na 0.44 [Mn 0.44 Ti 0.56 ]O 2 (molar ratio, NO 2 BF 4 : Na 0.44 [Mn 0.44 Ti 0.56 ]O 2 =0.22:1) was added to the resulting solution. The slurry was stirred overnight at room temperature, filtered under vacuum and then finally washed several times with acetonitrile. Both electrode samples and powder samples were then pressed onto conducting carbon tapes and loaded into our special sample transfer chamber inside the argon glove box. The sample transfer chamber was sealed and mounted directly onto the ultra-high vacuum XAS characterization chamber to avoid any air exposure effects [52] . sXAS was performed at Beamline 8.0.1 of the Advanced Light Source (ALS) in LBNL [53] . The undulator and spherical grating monochromatic supply a linearly polarized photon beam with resolving power up to 6,000. The experimental energy resolution is about 0.15 eV. Experiments were performed at room temperature and with the linear polarization of the incident beam 45° to sample surfaces. Data were collected in surface-sensitive total electron yield mode with the probing depth around several nanometers. All the spectra have been normalized to the beam flux measured by the upstream gold mesh. STEM imaging A JEM-ARM200F STEM fitted with a double aberration-corrector for both probe-forming and imaging lenses is used to perform HAADF imaging, which was operated at 200 KV. The convergence angle was 25 mrad and the angular range of collected electrons for HAADF imaging is about 70–250 mrad. Atomic resolution STEM-EELS line scanning was performed vertical throughout the interfaces, providing an energy resolution of 0.4 eV. Ti L2,3 and Mn L2,3 edges were acquired simultaneously and a suitable energy dispersion of 0.25 eV per pixel was selected. Electrochemistry The working electrode was prepared by spreading the slurry of the active materials (75 wt.%), acetylene black (15 wt.%) and the polyvinylidene fluoride (10 wt.%) binder on Al foil. The working electrodes were dried at 100 °C under vacuum for 10 h. The electrolyte is 1 M NaClO 4 in ethylene carbonate (EC)/diethyl carbonate (DEC) (4:6 in volume). The coin-type (CR2032) cells were assembled with pure sodium foil as the counter electrode, and a glass fibre as the separator in an argon-filled glove box. The charge and discharge measurements were carried out on a Land BT2000 battery test system in voltage ranges of 1.5–3.9 V and 1.8–2.8 V under room temperature. A three-electrode electrochemical cell was used for the discharge–charge tests in Na 2 SO 4 aqueous electrolytes (pH=13.5). The working electrode was prepared by mixing active material, acetylene black and polytetrafluoroethylene (PTFE) binder together in a 7:2:1 mass ratio and then pressing into nickel foam. A SCE/saturated KCl (RE-6, BASInc.) and platinum electrode were used as the reference and counter electrodes, respectively. Galvanostatic charge–discharge tests were carried out with a cycler (NAGANO BTS-2004W) at a constant current density. The full cells were charged and discharged between the voltage range of −0.6 to 0 V versus SCE at various current C-rates (2C current rate corresponds to 100 mA g −1 ). DFT calculations First-principles calculations are conducted based on the spin-polarized generalized gradient approximation (GGA) using the Perdew-Burke-Ernzerhof exchange-correlation parameterization to DFT [54] . A plane-wave basis set and the projector-augmented wave method, which is implemented in the Vienna ab initio simulation package [55] , was used. Hubbard parameter (GGA+U) was applied to correct the incomplete cancelation of the self-interaction effect of GGA method [56] , [57] . U value of 4.9 and 2.5 eV were used for Mn and Ti, respectively, and J value of 1 eV was applied for both elements. All calculations are conducted in × b × 4c super cells for 72 formula units. A plane-wave basis with a kinetic energy cutoff of 500 eV was used and reciprocal space k-point meshes of 3 × 1 × 3 were used to convince convergence within 1 meV per formula unit. All structures are calculated in a ferromagnetic ordering, since ant ferromagnetic arrangements are reported to be higher energies. To calculate exact formation energy and voltage, electrostatic energy of all possible configurations of composition by Ewald summation technique was calculated, and 30 structures of lowest electrostatic energy were collected in each composition. These structures were used as an input for first-principle calculation. How to cite this article: Wang, Y. et al. Ti substituted tunnel-type Na 0.44 MnO 2 oxide as a negative electrode for aqueous sodium-ion batteries. Nat. Commun. 6:6401 doi: 10.1038/ncomms7401 (2015).